Rapid and quantitative one-pot synthesis of sequence-controlled polymers by radical polymerization A long-standing challenge in polymer chemistry has been to prepare synthetic polymers with not only well-defined molecular weight, but also precisely controlled microstructure in terms of the distribution of monomeric units along the chain. Here we describe a simple and scalable method that enables the synthesis of sequence-controlled multiblock copolymers with precisely defined high-order structures, covering a wide range of functional groups. We develop a one-pot, multistep sequential polymerization process with yields >99%, giving access to a wide range of such multifunctional multiblock copolymers. To illustrate the enormous potential of this approach, we describe the synthesis of a dodecablock copolymer, a functional hexablock copolymer and an icosablock (20 blocks) copolymer, which represents the largest number of blocks seen to date, all of very narrow molecular weight distribution for such complex structures. We believe this approach paves the way to the design and synthesis of a new generation of synthetic polymers. Biopolymers, such as proteins and nucleic acids, are defined by their highly specialized functions that arise from their perfectly controlled primary structures, that is, sequence regulation of repeat units and/or functionalities along the polymer backbone. This remarkable control at the molecular scale is particularly important for proteins, as it directs the folding of a single peptide chain into a precise tertiary three-dimensional structure and imbues the protein with its highly specific activity. One of the major challenges of modern chemistry is to synthetically mimic such high structural sequence specificity and to achieve the control required using a chemically efficient and easily scalable process. Although considerable progress has been made, for instance, through the establishment of solid-phase peptide synthesis [1] and native chemical ligation [2] , as well as through advances in genetic engineering (the programing of sequences of natural and non-canonical amino acids into bacterially derived peptides) [3] and artificial advanced template-based syntheses such as enzyme-free DNA translation [4] or using molecular machines [5] , none of these approaches reported to date are applicable to the synthesis of large amounts of material as required for applications. Indeed, chemical syntheses to date rely on complicated multistep protocols and processes that have very limited versatility; even what many consider the most promising approach, genetic engineering, has an inherent synthetic bottleneck as each peptide obtained relies on the previous highly specific synthesis of another sequence-defined polymer, that is, the coding DNA, by some means (for example, solid-phase synthesis). Nature’s precision in regulating monomer sequences also remains unmatched in non-natural macromolecules [6] , [7] , [8] , [9] , [10] . Among the various examples of sequence-regulated synthetic macromolecules, block copolymers exhibiting a large number and type of functional sequences – that is, multiblock copolymers—are unique and original structures that exhibit a type of primary structure (although the sequence control is typically limited by the monomer distribution within each block). Despite their promises, these structures have to date been limited to only a few blocks, with relatively broad molecular weight distribution (typically>1.5) and their synthesis typically requires a demanding process (low conversion, purification between each block formation and so on). However, as their synthesis is much more scalable than the various processes described above, the ability to create multiblock copolymers with a wide range of sequences would enable the creation of a completely new class of materials, the functionality of which can be designed ‘on demand’. For instance, these sequence-defined architectures could mimic the tertiary structure of proteins by folding into 3D structures through intramolecular interactions between specifically designed sequences, for example, to form unimolecular nanoparticles with enhanced catalytic activity and specificity, thus mimicking enzymes [11] , or to generate even more complex architectures such as unimolecular nanopores, which mimic transmembrane channel proteins [12] . A strategy for the simple synthesis of multiblock copolymers of various types would also enable the generation of precisely tailored materials through self-assembly, with unparalleled control over nanoscale-domain geometry, packing symmetry and chemical composition [13] . This report describes the first example of a synthetic route that provides multiblock copolymers combining precisely defined and high-order structures of well-defined molecular weight distributions (dispersity<1.4) with a wide range of functional groups and simple as well as scalable syntheses. We have developed a one-pot, sequential polymerization process with yields of over 99%, thereby giving access to a wide range of well-defined multifunctional multiblock copolymers. This process is based on a radical polymerization proceeding by degenerative transfer, under non-stringent reaction conditions, thus rendering the approach amenable to scale-up. To illustrate the enormous potential of this approach, we describe the synthesis of a dodecablock containing repetitions of four different sequences of ten units each, a hexablock containing repetitions of five different sequences of 5–25 units each and a multiblock copolymer with the world’s highest number of blocks so far—an icosablock (20 blocks) copolymer of exceptionally narrow molecular weight distribution, containing repetitions of three different sequences of on average three units each. Synthetic route to multiblock copolymer We focused this study on acrylamide derivatives, a monomer family with high k p (high k p /( k t ) 1/2 , k p and k t are the propagation and termination rate coefficients, respectively) and one that provides access to a wide range of functional groups through amide bonds. Our first target was a dodecablock copolymer with a degree of polymerization (DP) of 10 for each block comprising four different monomers, based on three monomer sequences of N , N -dimethylacrylamide (DMA), 4-acryloylmorpholine (NAM), N , N -diethylacrylamide (DEA) and N -isopropylacrylamide (NIPAM) ( Fig. 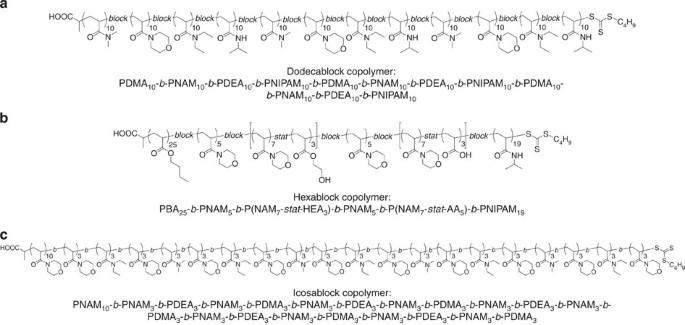Figure 1: Structure of the multiblock copolymers. The multiblock copolymers are synthesized in a one-pot multistep reversible addition-fragmentation chain transfer (RAFT) process. (a) Structure of the dodecablock copolymer synthesized in dioxane at 65 °C with AIBN as initiator and for 24 h per block. (b) Structure of the hexablock copolymer synthesized in dioxane at 65 °C with AIBN as initiator and for 24 h per block. (c) Structure of the icosablock copolymer synthesized in water at 70 °C with VA-044 as initiator allowing 2h per block. 1a , run 1; Table 1 ). The initial conditions were designed for 65 °C in dioxane, and preliminary experiments revealed that an optimal monomer concentration of 2 M for the first block enables rapid polymerization and workable solution viscosity. 2-(((Butylthio)carbonothiolyl)thio)propanoic acid and 2,2′-azobis(2-methylpropionitrile) (AIBN) were chosen as chain trasnfer agent (CTA) and radical initiator, respectively, resulting in consumption of ~81% of the initiator during the polymerization time of 24 h ( Supplementary Table S1 ; after each 24 h period, monomer/initiator/dioxane are added). High overall monomer conversions for each block (~97–100%) were confirmed by 1 H NMR spectroscopy ( Fig. 2a ; Supplementary Table S2 ). Analysis of the molecular weight distributions by size-exclusion chromatography (SEC) revealed monomodal distributions with a clear shift to higher molecular weights after each monomer addition ( Fig. 2b ). Some low-molecular-weight tailing was observed after each block extension, ascribed to the accumulation of initiator-derived chains, dead polymer chains and possible interactions of the multiblock copolymer with the SEC column, leading to a dispersity continuously increasing from 1.2 to 1.6 ( Fig. 2c ; Supplementary Table S2 ). As in all systems based on a degenerative transfer mechanism, the number of dead chains is dictated by the number of chains originating from the radical initiator and the number of living chains corresponds to the initial number of CTA. In this system, after 12 cycles, the theoretical fraction of living chains is ~90% (run 1, Table 1 ), and this high degree of livingness is clearly illustrated experimentally by the good control over the molecular weight distributions despite applying as many as 12 cycles ( Fig. 2b ). Further evidence is obtained from matrix-assisted laser desorption/ionization Fourier transform ion cyclotron resonance mass spectrometry (MALDI-FT-ICR MS) analysis, which shows that the number of dead chains and initiator-derived chains is below the detection limit for the first two cycles ( Supplementary Figs S1–S3 ; Supplementary Tables S3 and S4 ; spectra of the subsequent blocks cannot be quantitatively analysed due to overlapping). Although the evolution of the experimental molecular weight ( M n,SEC ) with the number of blocks ( Fig. 2c ) cannot be plotted accurately, as blocks of different nature considerably affect the hydrodynamic volume of the multiblock copolymer, a linear evolution is observed and confirms that the number of initiator-derived polymer chains is still negligible in comparison to the total number of CTA initially introduced. The very high conversions of each block extension and the one-pot nature of this reaction led to 8 g of a dodecablock containing three repetitions of four different sequences of an average of ten units each with a total molecular weight ( M n,LS ) of 15,200 g mol −1 (absolute molecular weight determined by light scattering (LS), close to the theoretical molecular weight of 14,400 g mol −1 ), a scale that is several orders of magnitude larger than that of any other sequence-specific polymer synthesis reported so far. Figure 1: Structure of the multiblock copolymers. The multiblock copolymers are synthesized in a one-pot multistep reversible addition-fragmentation chain transfer (RAFT) process. ( a ) Structure of the dodecablock copolymer synthesized in dioxane at 65 °C with AIBN as initiator and for 24 h per block. ( b ) Structure of the hexablock copolymer synthesized in dioxane at 65 °C with AIBN as initiator and for 24 h per block. ( c ) Structure of the icosablock copolymer synthesized in water at 70 °C with VA-044 as initiator allowing 2h per block. Full size image Table 1 Summary of the multiblock copolymers synthesized in this study. 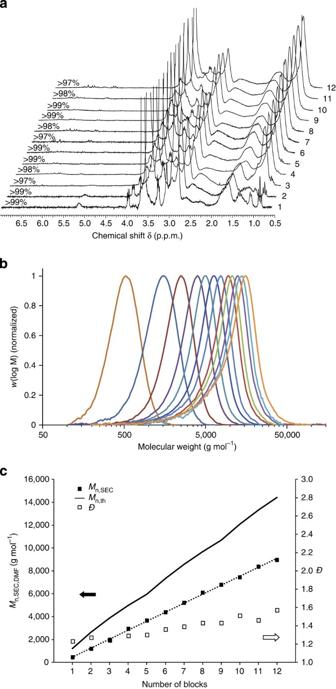Figure 2: Data analysis for the dodecablock copolymer 1a. The sample is obtained by iterative RAFT polymerization. (a)1H NMR spectra (CDCl3, 300 MHz) showing the monomer conversion for each block after 24 h of iterative RAFT polymerization. (b) Molecular weight distributions for successive block extensions of the dodecablock copolymer in dioxane at 65 °C with AIBN as initiator (24 h per block). (c) Evolution of number average molecular weights and dispersities with the number of blocks for the preparation of the dodecablock copolymer 1a. The black line represents the theoretical molecular weight calculated without taking account of the initiator-derived term:Mn,th=[Monomer]0×p×MMonomer/[CTA]0+MCTA. Full squares represent the experimental molecular weight from SEC. Empty squares represent the dipersities from SEC. Full size table Figure 2: Data analysis for the dodecablock copolymer 1a. The sample is obtained by iterative RAFT polymerization. ( a ) 1 H NMR spectra (CDCl 3 , 300 MHz) showing the monomer conversion for each block after 24 h of iterative RAFT polymerization. ( b ) Molecular weight distributions for successive block extensions of the dodecablock copolymer in dioxane at 65 °C with AIBN as initiator (24 h per block). ( c ) Evolution of number average molecular weights and dispersities with the number of blocks for the preparation of the dodecablock copolymer 1a. The black line represents the theoretical molecular weight calculated without taking account of the initiator-derived term: M n,th =[Monomer] 0 × p × M Monomer /[CTA] 0 + M CTA . Full squares represent the experimental molecular weight from SEC. Empty squares represent the dipersities from SEC. Full size image Preparation of highly functional multiblock copolymer To further demonstrate the level of structural intricacy that can be achieved easily via our approach, another multiblock copolymer was targeted that exhibits a unique level of complexity for a sequential block copolymer ( Fig. 1b , run 2; Table 1 ). A hexablock copolymer was designed with an initial hydrophobic block of poly( n -butyl acrylate), poly( n BA), comprising 25 units followed by two hydrophilic and functional statistical segments of NAM/hydroxyl ethyl acrylate (HEA) (introducing a hydroxyl group) and NAM/acrylic acid (AA) (introducing a carboxylic acid). Between each block, a very short sequence of five NAM units was programmed as an inert backbone. The final block was built from 19 units of NIPAM, to yield an amphiphilic functional multiblock copolymer ( Supplementary Table S5 ). Again, high monomer conversion ( Fig. 3a ) and very good control of the molecular weight distribution was achieved ( Fig. 3b ; Supplementary Table S6 ). The low-molecular-weight tailing for the last two blocks is enhanced by the interactions of the acrylic acid units (fifth block) and poly(NIPAM) (sixth block) with the SEC columns. Theory dictates that the final multiblock copolymer comprises 95% living chains, consistent with the low dispersity of 1.36 as well as the absence of initiator-derived polymer chains observed for the first block by MALDI-FT-ICR ( Supplementary Fig. S4 ; Supplementary Table S7 ). This hexablock copolymer, with a total molecular weight ( M n,LS ) of 11,000 g mol −1 (absolute molecular weight, close to the theoretical molecular weight of 9,400 g mol −1 ), was subsequently assembled in aqueous solution. Although a multiblock copolymer with a hydrophobic:hydrophilic segment ratio of 1:2 is expected to form spherical micelles in water at room temperature [13] (average of 25 units of n BA, 20 units of segmented NAM, HEA and AA and 19 units of NIPAM), dynamic light scattering (DLS) analyses reveals the presence of unimers only (sizes of 2–3 nm), suggesting that the multiblock structure affects the amphiphilic properties of the polymer ( Supplementary Fig. S5 ). On a temperature increase to 80 °C, the poly(NIPAM) block undergoes a hydrophilic-to-hydrophobic transition, to form a hydrophobic–hydrophilic–hydrophobic segmented chain, which is then observed to assemble into small particles of 30 nm diameter ( Supplementary Fig. S5 ). As this type of ABA amphiphilic structures are expected to form flower-like micelles in water [13] , the remarkable sequence control we obtain over the hexablock structure may enable the display of hydroxyl functionalities (poly(NAM- stat -HEA) block) and carboxylic acid functionality (poly(NAM- stat -AA) block) on the corona of the micelle. 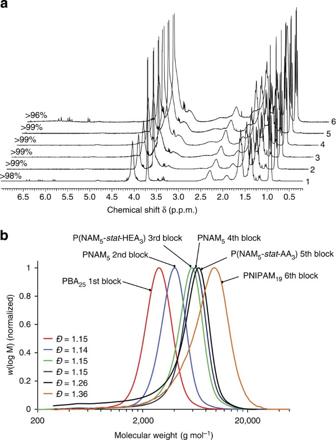Figure 3: Data analysis for the hexablock copolymer 1b. The sample is obtained by iterative RAFT polymerization. (a)1H NMR spectra (CDCl3, 300 MHz) showing the monomer conversion for each block after 24 h of iterative RAFT polymerization. (b) Molecular weight distributions for successive block extensions of the hexablock copolymer 1b in dioxane at 65 °C with AIBN as initiator (24 h per block). Figure 3: Data analysis for the hexablock copolymer 1b. The sample is obtained by iterative RAFT polymerization. ( a ) 1 H NMR spectra (CDCl 3 , 300 MHz) showing the monomer conversion for each block after 24 h of iterative RAFT polymerization. ( b ) Molecular weight distributions for successive block extensions of the hexablock copolymer 1b in dioxane at 65 °C with AIBN as initiator (24 h per block). Full size image Pushing the limit of the radical process Having demonstrated the viability of our approach, we embarked on further tuning of the system to increase the polymerization rate and the fraction of living chains, while keeping to near complete monomer conversions. In this system, the fraction of living chains depends on the total amount of initiator decomposed during the polymerization and not on the concentration of propagating radicals as depicted in equation (1): where L is the number fraction of living chains, [CTA] 0 and [ I ] 0 are the initial concentrations of CTA and initiator, respectively. The term ‘2’ means that one molecule of azo initiator gives two primary radicals with a certain efficiency f (taken as 0.5 in this study). k d is the decomposition rate coefficient of the initiator. The term 1− f c /2 represents the number of chains produced in a radical–radical termination event with f c the coupling factor ( f c =1 means 100% bimolecular termination by combination, f c =0 means 100% bimolecular termination by disproportionation). In this study, a value of f c =0 was used. This dependance is a consequence of all chains generated by the initiator eventually terminating (consider a scenario where k t is extraordinarily high – this would not cause an increase in the fraction of dead chains, it would merely limit the final conversion reached). It follows that it is possible to increase the polymerization rate without a concomitant loss in livingness by choosing a radical initiator that decomposes more rapidly, while still generating the same cumulant number of radicals over the course of the polymerization. For this purpose, the initiator 2,2′-azobis[2-(2-imidazolin-2-yl)propane]dihydrochloride (VA-044, Fig. 4 ) was employed (~95% of VA-044 is decomposed in 2 h, relatively similar to 81% of AIBN in 24 h). As the solvent choice may also significantly affect rate constants, we were interested in the use of water, which in addition to being environmental friendly and allowing the production of water-soluble macromolecules, is also known to increase k p of acrylamide monomers [14] . To further test the system, we focused on multiblock copolymers comprising a large number of very short blocks (average of three monomer units), as in all living radical polymerization (LRP) systems, targeting low degrees of polymerization leads to a greater number of chains and, therefore, a higher fraction of chains with an active chain end. A poly(NAM) of DP 10 (PNAM 10 ) was used as a water-soluble macroCTA, followed by alternating segments of PNAM 3, PDMA 3 , PNAM 3 and PDEA 3 (PNAM 3 to decrease the interaction of the two segments PDMA 3 and PDEA 3 on the SEC column), the whole sequence was repeated five times, in H 2 O/70 °C/VA-044 (2 h per block), to form a 20-block copolymer ( Figs 1c and 4a ; Supplementary Tables S8 and S9 ). Remarkable control was achieved for such a complex and demanding architecture. The very high robustness of the process allowed us to stop the reaction after five successive blocks, keep the polymerization mixture overnight in the fridge, then restart the synthesis for five new blocks, and so on over 4 days to reach a 20-block copolymer with ~98–99% monomer conversion for each block ( Fig. 5a ; Supplementary Table S10 ). Mass spectroscopy analysis ( Fig. 6 ; Supplementary Figs S6–S13 , Supplementary Tables S11–S14 ) of the first five blocks shows a very high end-group retention and one can detect neither dead chains, nor initiator-derived chains (spectra beyond five blocks cannot be quantitatively analysed due to overlapping). The evolution of the chromatograms in SEC-THF shows 20 successful block extensions ( Fig. 5b ; Supplementary Figs S14 and S15 ), leading to a copolymer of M n 12,100 g mol −1 (absolute molecular weight, close to the theoretical M n of 9,200 g mol −1 considering the analytical error due to high number of the various functionalities) containing repetitions of three different sequences of three units each with dispersity remaining amazingly low for such a complex structure, that is, between 1.10 and 1.36 ( Fig. 5c ; Supplementary Table S10 ). 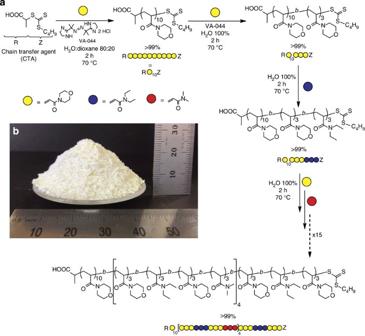Figure 4: Synthesis of multiblock copolymers by the reversible addition-fragmentation chain transfer mechanism. (a) Schematic representation of the synthesis of the icosablock copolymer 1c used as an example. (b) The image shows the total amount of product obtained after 20 chain extensions (after precipitation in diethyl ether). Figure 4: Synthesis of multiblock copolymers by the reversible addition-fragmentation chain transfer mechanism. ( a ) Schematic representation of the synthesis of the icosablock copolymer 1c used as an example. ( b ) The image shows the total amount of product obtained after 20 chain extensions (after precipitation in diethyl ether). 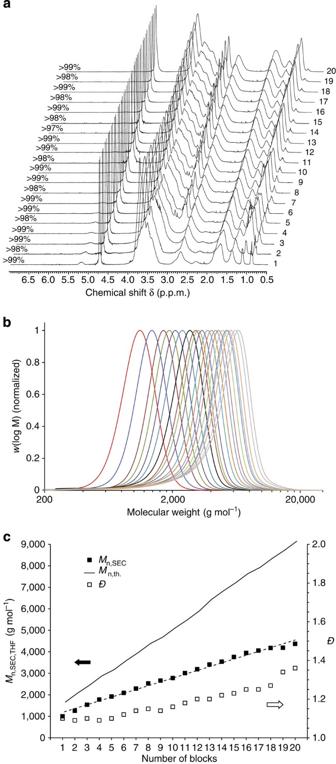Figure 5: Data analysis for the icosablock copolymer 1c. The sample is obtained by iterative RAFT polymerization. (a)1H NMR spectra (D2O, 300 MHz) showing the monomer conversion for each block after 2 h of iterative RAFT polymerization. (b) Molecular weight distributions for successive block extensions of the icosablock copolymer in water at 70 °C with VA-044 as initiator (2 h per block). (c) Evolution of number average molecular weights and dispersities with the number of blocks for the preparation of the icosablock copolymer 1c. The black line represents the theoretical molecular weight calculated without taking account of the initiator-derived term:Mn,th=[Monomer]0×p×MMonomer/[CTA]0+MCTA. Full squares represent the experimental molecular weight from SEC. Empty squares represent the dipersities from SEC. Full size image Figure 5: Data analysis for the icosablock copolymer 1c. The sample is obtained by iterative RAFT polymerization. ( a ) 1 H NMR spectra (D 2 O, 300 MHz) showing the monomer conversion for each block after 2 h of iterative RAFT polymerization. ( b ) Molecular weight distributions for successive block extensions of the icosablock copolymer in water at 70 °C with VA-044 as initiator (2 h per block). ( c ) Evolution of number average molecular weights and dispersities with the number of blocks for the preparation of the icosablock copolymer 1c. The black line represents the theoretical molecular weight calculated without taking account of the initiator-derived term: M n,th =[Monomer] 0 × p × M Monomer /[CTA] 0 + M CTA . Full squares represent the experimental molecular weight from SEC. Empty squares represent the dipersities from SEC. 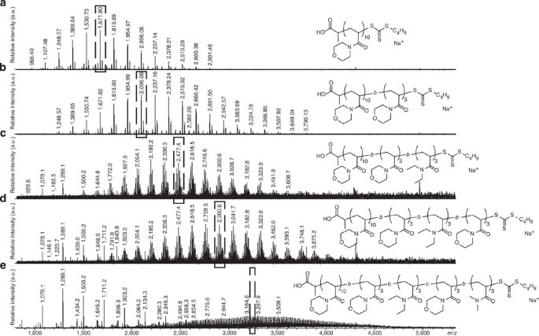Figure 6: Mass spectra of the first five blocks for the icosablock copolymer 1c. The sample is obtained by iterative RAFT polymerization. (a) Mass spectrum of the first block PNAM10(cationized Na+) obtained after 2 h RAFT polymerization.The highlighted peaks correspond to the structure shown. (b) Mass spectrum of the diblock copolymer PNAM10-b-PNAM3(cationized Na+) obtained after chain extension of the PNAM10with the monomer NAM. The highlighted peaks correspond to the structure shown. (c) Mass spectrum of the triblock copolymer PNAM10-b-PNAM3-b-PDEA3(cationized Na+) obtained after chain extension of the diblock PNAM10-b-PNAM3with the monomer DEA. The highlighted peaks correspond to the structure shown. (d) Mass spectrum of the tetrablock copolymer PNAM10-b-PNAM3-b-PDEA3-b-PNAM3(cationized Na+) obtained after chain extension of the triblock PNAM10-b-PNAM3-b-PDEA3with the monomer NAM. The highlighted peaks correspond to the structure shown. (e) Mass spectrum of the pentablock copolymer PNAM10-b-PNAM3-b-PDEA3-b-PNAM3-b-PDMA3(cationized Na+) obtained after chain extension of the tetrablock PNAM10-b-PNAM3-b-PDEA3-b-PNAM3with the monomer DMA. The highlighted peaks correspond to the structure shown. Full size image Figure 6: Mass spectra of the first five blocks for the icosablock copolymer 1c. The sample is obtained by iterative RAFT polymerization. ( a ) Mass spectrum of the first block PNAM 10 (cationized Na + ) obtained after 2 h RAFT polymerization.The highlighted peaks correspond to the structure shown. ( b ) Mass spectrum of the diblock copolymer PNAM 10 - b -PNAM 3 (cationized Na + ) obtained after chain extension of the PNAM 10 with the monomer NAM. The highlighted peaks correspond to the structure shown. ( c ) Mass spectrum of the triblock copolymer PNAM 10 - b -PNAM 3 - b -PDEA 3 (cationized Na + ) obtained after chain extension of the diblock PNAM 10 - b -PNAM 3 with the monomer DEA. The highlighted peaks correspond to the structure shown. ( d ) Mass spectrum of the tetrablock copolymer PNAM 10 - b -PNAM 3 - b -PDEA 3 - b -PNAM 3 (cationized Na + ) obtained after chain extension of the triblock PNAM 10 - b -PNAM 3 - b -PDEA 3 with the monomer NAM. The highlighted peaks correspond to the structure shown. ( e ) Mass spectrum of the pentablock copolymer PNAM 10 - b -PNAM 3 - b -PDEA 3 - b -PNAM 3 - b -PDMA 3 (cationized Na + ) obtained after chain extension of the tetrablock PNAM 10 - b -PNAM 3 - b -PDEA 3 - b -PNAM 3 with the monomer DMA. The highlighted peaks correspond to the structure shown. Full size image Our approach is based on implementing a degenerative transfer mechanism in a radical polymerization ( Fig. 4 ), tuning the reaction conditions such that the polymerization proceeds to full conversion, in a reasonable time, whilst keeping an unprecedented level of control and providing large quantities of product. Radical processes are always plagued by radical termination reactions, for example, bimolecular termination or irreversible transfer reactions involving propagating radicals, resulting in polymeric chains of uncontrolled structure. In a degenerative transfer polymerization, two types of chains are generated: (i) chains formed via the degenerative transfer step (desired chains), and (ii) chains formed by radical termination reactions (undesired chains). Importantly, the number of chains originating from termination reactions in a degenerative transfer polymerization can be readily predicted from the number of radical initiators consumed, which is based on the initial stoichiometry. In a process based on degenerative transfer, radicals (typically generated from a radical initiator) are transferred between polymer chains via a CTA, resulting in periodic activation/deactivation of chains. During the active state of a given chain (that is, when it acts as propagating radical), monomer units can be added. This is followed by its deactivation through reaction with the CTA and the subsequent transfer of the radical to a neighbouring chain via the CTA. When all the monomer has been consumed, the system contains chains carrying a CTA, so-called living chains. These are all of near-equal length and their number equals the initial number of CTAs. In addition, there are chains created continuously throughout the polymerization from the radicals generated by the initiator decomposition. These chains will undergo termination reactions, have uncontrolled length and cannot be extended as they do not possess the CTA living group at their ω-chain end. However, their number can be predicted based on the number of decomposed free radical initiators. Consequently, the number of dead chains is reduced when decreasing the amount of initiator used. Typically, a reduced initiator concentration (for example, reducing the amount of initiator at constant volume) is expected to lead to a lower polymerization rate. However, the rate can also be controlled by the variation of other independent parameters, including monomer concentration, temperature, solvent and so on. This feature thus enables one to independantly tune the system in terms of polymerization rate and fraction of living chains via an appropriate choice of initiator concentration and general polymerization conditions. Although several radical polymerization systems are based on the concept of degenerative transfer [15] —for instance reversible addition-fragmentation chain transfer (RAFT) polymerization, organotellurium-mediated radical polymerization and iodide-mediated radical polymerization—the ability to maintain a high fraction of living chains by the independent tuning of both the number of living chains and of the rate has been overlooked. It is important to stress that in this regard degenerative transfer LRP systems are distinctly different from other LRP systems, which operate based on reversible termination, such as nitroxide-mediated radical polymerization and atom transfer radical polymerization—in degenerative transfer systems, bimolecular termination or irreversible transfer reactions involving propagating radicals do not lead to loss of living chain ends. In this work, we have used the RAFT process because of its versatility in terms of monomer choice, polymer architectures and reaction conditions [16] , [17] , [18] . The ability to tune rate/fraction of living chains independently in combination with the high tolerance to monomer functionality of the RAFT process have enabled us to develop a synthetic pathway to multiblock copolymers with far superior control over molecular weight distribution as well as a higher number of sequences and functionalities than ever reported before [19] , [20] , [21] . To achieve complete monomer consumption and a very high fraction of living chains during the synthesis of each block, a precise understanding of the kinetics governing the polymerization process is required. The rate of propagation is given by equation (2): where R p is the rate of propagation, k p the propagation rate coefficient, [ M ] the monomer concentration, f the initiator efficiency, k d the decomposition rate coefficient of the initiator, [ I ] 0 the initial initiator concentration and k t the termination rate coefficient. The polymerization rate increases with: (i) increasing temperature; (ii) an increase in k p /( k t ) 1/2 , which is directly linked to the choice of monomer; (iii) the monomer concentration ([ M ]) and (iv) the concentration and rate of decomposition of the radical initiator. Assuming RAFT end groups are not consumed in side reactions, the final number of living chains is equal to the number of RAFT agents initially introduced. It follows that the chain end retention is perfect, but the fraction of living chains decreases due to the increase in the number of chains derived from the radical initiator. The key point in our approach is to tune the conditions such that the polymerization proceeds to full conversion in a reasonable time and to use a very low ratio of initiator-to-RAFT agent. In conclusion, we have established a process that enables synthesis of large amounts of highly complex multiblock copolymers, with each block reaching near to full conversion in one-pot, with no purification steps. We illustrate the versatility of our approach with three proof-of-concept examples, a dodecablock, a functional amphiphilic hexablock and an icosablock copolymer. Importantly, although the approach is illustrated for RAFT polymerization, it applies equally well to all processes based on degenerative transfer. The method highlights a hitherto overlooked key feature of degenerative transfer LRP systems, namely the fact that the extent of bimolecular termination can be controlled via the initiator concentration. The access to such a high level of complexity in polymer microstructure via such a manageable synthetic route (quantitative conversion for each block, no purification needed, no stringent reaction conditions, fast—2 h—polymerization times) offers new perspectives for the design of new families of highly functional polymers. Materials Tetrahydrofuran (THF, Ajax Finechem, 99%), N , N -dimethylformamide (DMF; Merck, HPLC-grade), 2,2′-Azobis[2-(2-imidazolin-2-yl)propane]dihydrochloride (VA-044, Wako) were used without further purification. Milli-Q water. 1,4-Dioxane (Sigma-Aldrich, ≥99%) was distilled under reduced pressure before use. Butyl acrylate (BA; Sigma-Aldrich, ≥99%), 2-hydroxyethyl acrylate (HEA, Sigma-Aldrich, ≥96%), N , N -dimethylacrylamide (DMA, Sigma-Aldrich, 99%), were filtered through a basic aluminium oxide (activated, basic, Brockmann I, standard grade, ~150 mesh, 58A) column before use, to remove the radical inhibitor. N -isopropylacrylamide (NIPAM; Sigma-Aldrich, 97%) was used after purification by recrystallization in n -hexane. Acrylic acid (AA; Sigma-Aldrich, 99%), 4-acryloylmorpholine (NAM, Sigma-Aldrich, 97%), N,N -diethylacrylamide (DEA) were purified by vacuum distillation. All polymerizations were carried out under an argon atmosphere. 2,2′-Azobis(2-methylpropionitrile) (AIBN) was recrystallized twice from methanol and dried under reduced pressure before use. The RAFT agent, 2-(((Butylthio)carbonothiolyl)thio)propanoic acid was received from Dulux Group Australia and used as received. NMR spectroscopy 1 H NMR spectra were recorded on a Bruker Avance 300 spectrometer (300 MHz) at 27 °C in chloroform- d (CDCl 3 ) or D 2 O. The delay time (d1) was set to 2 s. Chemical shift values ( δ ) are reported in p.p.m. TMS was used as internal standard for calibrating chemical shifts in CDCl 3 . In D 2 O, the residual proton signal of the solvent was used as internal standard ( δ H =4.79 p.p.m.). Size-exclusion chromatography Molar mass distributions were measured either on a Shimadzu LC-20AD or on an Agilent GPC50 liquid chromatography system. The Shimadzu LC-20AD liquid chromatography system used a Jordi Gel DVB 500Å guard column (50 × 7.8 mm) followed by two PL gel, 5 μm, MIXED-C (300 × 7.5 mm). THF was used as eluent at 1.0 ml min −1 , at 40 °C and with 0.5 vol% toluene (flow rate marker). Polystyrene standards were used to calibrate the SEC system. Analyte samples contained toluene (0.5 vol%) as the flow rate marker and were filtered through a polytetrafluoroethylene (PTFE) membrane with a 0.2-μm pore before injection (100 μl). Respectively, experimental molar mass ( M n,SEC ) and dispersity ( Ð ) values of synthesized polymers were determined by conventional calibration using ASTRA for Windows software (Version 6.90.08) with known RI detector calibration constant. The Agilent GPC50 liquid chromatography system used a Polar Gel-M guard column (50 × 7.5 mm) and two Polar Gel-M columns (300 × 7.5 mm). DMF+0.1% LiBr was used as eluent at 0.7 ml min −1 at 50 °C. Polystyrene standards were used to calibrate the SEC system. Analyte samples contained water (0.5 vol%) as the flow rate marker and were filtered through a polytetrafluoroethylene (PTFE) membrane with 0.2 μm pore before injection (100 μl). Respectively, experimental molar mass ( M n,SEC ) and dispersity ( Ð ) values of synthesized polymers were determined by conventional calibration using Cirrus software with known RI detector calibration constant. Mass spectrometry Matrix-assisted laser desorption/ionization Fourier transform ion cyclotron resonance mass spectrometry (MALDI-FT-ICR MS) was performed using a Bruker Apex Qe 7T Dual ESI/MALDI-FT-ICR MS (Billerica MA) equipped with a Nd:YAG laser at 355 nm and 200 Hz at 20–40% laser power (100–200 μJ). The spectra were the sum of 800 shots, and an external mass calibration was used (PEG 600 and PEG 1,500 ). The samples were deposited onto a MTP AnchorChip plate and dried. Samples were prepared by dissolving the polymer in THF or a mixture CH 2 Cl 2 /MeOH (1/1:v/v) at a concentration of 10 g l −1 . The matrix was α-cyano-4-hydroxycinnamic acid (Sigma-Aldrich), used without further purification and dissolved in THF (10 g l −1 ). The salt was sodium iodide (NaI, Sigma-Aldrich) dissolved in MeOH at 10 g l −1 . For polymer solution in THF, matrix, salt and polymer solutions were mixed at a volume ratio of 2:10:1; for polymer solution in CH 2 Cl 2 /MeOH, matrix, salt and polymer solutions were mixed at a volume ratio of 1:1:1; then, 1 μl of the mixture was deposited onto the MALDI target before insertion into the ion source chamber. Dynamic light scattering Particle size measurements were carried out by DLS using a Malvern Instrument Zetasizer nano series instrument with a detection angle of 173°, where the intensity weighted mean hydrodynamic size ( Z -average) and the width of the particle size distribution were obtained from analysis of the autocorrelation function. Samples were filtered through a 0.45-μm membrane to ensure the minimization of dust and other particulates. At least 3–5 measurements at 25 °C were made for each sample with an equilibrium time of 5 min before starting measurement. The self-assembly of the hexablock copolymer was carried out via direct dissolution method by dissolving the multiblock copolymer (30 mg, 4.02 × 10 −6 mol) in Milli-Q water (30 ml) under vigorous stirring for 30 min. After sonication for 15 min, the solution was filtered through a 0.45-μm PTFE membrane filters and the diameter was measured by DLS. Multiblock copolymer preparation by RAFT polymerization A typical synthesis of the first block is the following: CTA, monomer, initiator and solvent are introduced in a flask equipped with a magnetic stirrer and seal with a rubber septum ( Supplementary Tables S1, S3 and S5 for the quantity of reagents needed for the three multiblock copolymers). The flask is degassed by bubbling argon through the solution for ca . 15 min, then the RAFT polymerization is performed in a thermostated oil bath at the desire temperature (65 or 70 °C). After 2 or 24 h, a sample is withdrawn from the polymerization medium using a degassed syringe for 1 H NMR, SEC and mass spectrometry analysis. Typical synthesis of the following blocks For the iterative chain extension, a further mixture of degassed monomer, initiator and solvent is added via gas-tight syringe to the polymerization medium and the polymerization mixture is allowed to polymerize at the same temperature (65 or 70 °C) for 24 h or 2 h with stirring ( Supplementary Tables S1, S3 and S5 for the quantity of reagents needed for the three multiblock copolymers). Before each new block, a sample is withdrawn from the polymerization medium using a degassed syringe for 1 H NMR, SEC and mass spectrometry analysis. This step is performed as many times as needed following the number of block desired. At any time before a new iterative chain extension, the polymerization can be stopped by storing the flask in the fridge until further chain extension. Determination of the monomer conversions For the dodecablock copolymer 1a, monomer conversions were determined by comparing the integral of the vinyl protons ( δ ~6.50–5.70 p.p.m.) of the monomer with the integral of the polymer backbone ( δ ~2.20–0.70 p.p.m.). For the hexablock copolymer 1b, the monomer conversions were determined by comparing the integral of the vinyl protons with the integral of the methyl protons ( δ ~1.10–0.70 p.p.m.) of the BA unit. For the icosablock copolymer 1c, the monomer conversions were calculated by comparing the integral of the vinyl protons with the integral of the RAFT agent methyl protons ( δ ~1.00–0.85 p.p.m.). Determination of the M n,th The number average theoretical molecular weight M n,th is determined with the equation (3): where [ M ] 0 , [CTA] 0 and [ I ] 0 are the initial concentrations of monomer, chain transfer agent and initiator, respectively, p is the monomer conversion determined by 1 H NMR, M M and M CTA are the molar masses of monomer and chain transfer agent, respectively. The term ‘2’ means that 1 molecule of azo initiator gives 2 primary radicals with a certain efficiency f (taken as 0.5 in this study). k d is the decomposition rate coefficient of the initiator. The term 1- fc /2 represents the number of chains produced in a radical–radical termination event with f c the coupling factor ( f c =1 means 100% bimolecular termination by combination, f c=0 means 100% bimolecular termination by disproportionation). In this study, The term relative to the initiator 2 f [ I ] 0 (1− e − k d t )(1- f c /2) is considered equal to 0 due to the negligible amount of initiator used in comparison with the amount of CTA. Determination of the number fraction of living chains L The number fraction of living chains is determined with the equation (2). For the system dioxane/AIBN/65 °C, we considered: k d(AIBN, 65 °C) =1.9254 × 10 −5 s −1 . For the system, H 2 O/VA-044/70 °C, we estimated k d(VA-044, 70 °C) =4.2995 × 10 −4 s −1 from theoretical k d(44 °C) =1.9254 × 10 −5 s −1 ; Ea=108,000 J mol −1 . How to cite this article: Gody, G. et al . Rapid and quantitative one-pot synthesis of sequence-controlled polymers by radical polymerization. Nat. Commun. 4:2505 doi: 10.1038/ncomms3505 (2013).